Bivalence Mn5O8with hydroxylated interphase for high-voltage aqueous sodium-ion storage Aqueous electrochemical energy storage devices have attracted significant attention owing to their high safety, low cost and environmental friendliness. However, their applications have been limited by a narrow potential window ( ∼ 1.23 V), beyond which the hydrogen and oxygen evolution reactions occur. Here we report the formation of layered Mn 5 O 8 pseudocapacitor electrode material with a well-ordered hydroxylated interphase. A symmetric full cell using such electrodes demonstrates a stable potential window of 3.0 V in an aqueous electrolyte, as well as high energy and power performance, nearly 100% coulombic efficiency and 85% energy efficiency after 25,000 charge–discharge cycles. The interplay between hydroxylated interphase on the surface and the unique bivalence structure of Mn 5 O 8 suppresses the gas evolution reactions, offers a two-electron charge transfer via Mn 2+ /Mn 4+ redox couple, and provides facile pathway for Na-ion transport via intra-/inter-layer defects of Mn 5 O 8 . Rechargeable aqueous electrochemical energy storage (EES) devices, especially ones using earth-abundant and non-toxic materials, have shown great promise for many applications owing to their high safety, low cost and environmental friendliness [1] . However, the thermodynamically stable potential window for aqueous EES has an intrinsic limit of 1.23 V, beyond which the hydrogen evolution reaction (HER) and oxygen evolution reaction (OER) occur. The evolved gas from electrolyte decomposition also severely deteriorates the electrode. A potential window of 1.23 V is too narrow for storage devices to achieve high energy and power performance. Extensive efforts have been made to break this limit on the potential window while retaining the benefits of aqueous energy storage systems. One approach is to adjust the pH of the electrolyte to suppress HER and/or OER [1] . An aqueous battery of 2.8 V was reported by using basic electrolyte in the anode compartment (to decrease HER potential following Nernst equation) and acidic electrolyte in the cathode compartment (to increase OER potential) [2] . A Li-ion-conductive membrane was therefore needed to separate two compartments with the drastic pH difference. Another approach to suppress gas evolution is through utilization of solid–electrolyte interphase (SEI). Such interphase is ion-conductive and but not electron-conductive, protecting the electrode (for example, Li anode) from direct contact with water [3] . Recently, Suo et al . reported a water-in-salt electrolyte, by dissolving concentrated Li-bis(trifluoromethane sulfonyl)imide salt in water. This electrolyte system introduces a desirable SEI that enables an aqueous Li-ion full cell operation at 2.3 V for more than 1,000 cycles [4] . Although these excellent works open up the opportunities for improving the potential window, the intrinsic limitation of the ionic conductivity in Li-ion-based aqueous systems has hindered high-rate performance of the cell, especially for the pseudocapacitive storage. Here we report a high-rate high-voltage aqueous Na-ion full cell system based on a surface hydroxylated Mn 5 O 8 electrode. As probed by synchrotron-based surface-sensitive soft X-ray spectroscopy (sXAS), an ice-like surface hydroxyl layer is formed after cycling. Density functional theory (DFT) calculations show that the interplay between the hydroxylated interphase and the unique bivalence (Mn 2+ 2 Mn 4+ 3 O 8 ) layered structure suppresses the HER and OER with a stable potential window of 3.0 V. The system exhibits a two-electron charge transfer via Mn 2+ /Mn 4+ redox couple, and provides facile pathway for Na-ion transport at high rate. The 3.0 V aqueous symmetric full cell exhibits a high energy density, 23 Wh kg −1 at a rate of 550 C, with nearly 100% coulombic efficiency and 85% energy efficiency after 25,000 charge–discharge cycles. Synthesis and characterizations of Mn 5 O 8 nanoparticles Mn 5 O 8 is the only bivalent manganese oxide that has a layered structure [5] . Although Mn 5 O 8 has abundant interlayer and intralayer defects for facile ionic transport, its capability for energy storage has rarely been reported. In this work, Mn 5 O 8 nanoparticles were synthesized by heating Mn 3 O 4 nanoparticles at 270 °C for 2 h in the open air. X-ray and neutron pair distribution function (PDF) analyses, shown in Fig. 1a,b , point to the formation of monoclinic Mn 5 O 8 ( Supplementary Tables 1 and 2 ), which consists of two-dimensional octahedral sheets of [Mn 3 4+ O 8 ] in the bc plane separated by Mn 2+ layers, giving a compositional formula of Mn 2+ 2 Mn 4+ 3 O 8 . Half of the Mn 4+ sites in the main octahedral sheets are not fully occupied, above and below these vacant sites are Mn 2+ sites ( Fig. 1c ). Apart from the major component Mn 5 O 8 , a small amount of Mn 3 O 4 is present as seen in both the X-ray diffraction ( Supplementary Fig. 1 ) and PDF analyses. Transmission electron microscopy (TEM) and scanning TEM showed that Mn 5 O 8 particles have an average size of 19 nm and possess a highly crystalline monoclinic structure ( Fig. 1d,e ) [5] . X-ray photoelectron spectroscopy (XPS) was used to analyse the surface of Mn 5 O 8 nanoparticles, where only manganese, oxygen, carbon and trace sodium signals can be detected without other surface residuals from synthesis and processing ( Supplementary Fig. 2 ). XPS data show that Mn 2+ and Mn 4+ valences in both 2p and 3s chemical states. The XPS spectra are fitted to Mn 3 s doublets, which are split by 5.7 eV (Mn 2+ ) and 4.5 eV (Mn 4+ ), respectively. The integrated intensity ratio of Mn 2+ and Mn 4+ is calculated to be around 1: 2, close to that of theoretical value from Mn 5 O 8 at near surface. 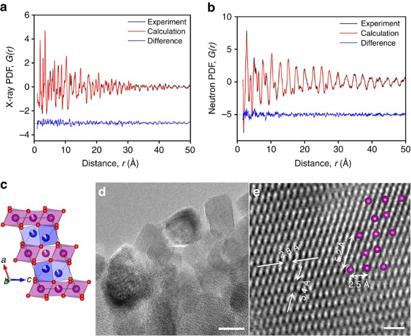Figure 1: Structure characterizations of Mn5O8nanoparticles. (a) X-ray and (b) neutron PDF analyses of Mn5O8nanoparticles. (c) Lattice structure of Mn5O8(purple: Mn4+; blue: Mn2+; red: O; white: probability of unoccupied site) obtained from PDF fitting; (d) TEM and (e) STEM images of Mn5O8nanoparticles (inset showed Mn5O8lattice (Mn only) along <010> direction). Scale bars, 20 nm (d) and 1 nm (e), respectively. Figure 1: Structure characterizations of Mn 5 O 8 nanoparticles. ( a ) X-ray and ( b ) neutron PDF analyses of Mn 5 O 8 nanoparticles. ( c ) Lattice structure of Mn 5 O 8 (purple: Mn 4+ ; blue: Mn 2+ ; red: O; white: probability of unoccupied site) obtained from PDF fitting; ( d ) TEM and ( e ) STEM images of Mn 5 O 8 nanoparticles (inset showed Mn 5 O 8 lattice (Mn only) along <010> direction). Scale bars, 20 nm ( d ) and 1 nm ( e ), respectively. 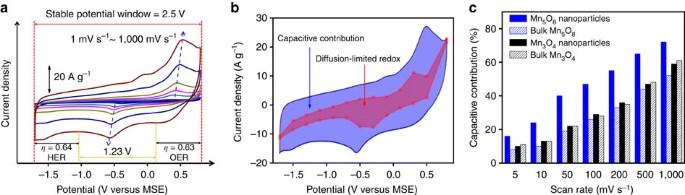Figure 2: Electrochemical measurements of Mn5O8electrodes in a half-cell. (a) CVs show a stable potential window of 2.5 V and large overpotential (η) towards HER and OER. (b) Electro-kinetics study of CV at 500 mV s−1. The contributions from capacitive process (blue) and diffusion-limited redox process (red) are shaded. (c) Capacitive contribution to the total charge stored at various scan rates in Mn5O8and Mn3O4nanoparticles and bulk materials. Full size image Electrochemical studies of Mn 5 O 8 Figure 2a shows the cyclic voltammetry (CV) curves of the Mn 5 O 8 -based electrodes. The Mn 5 O 8 material was mixed with carbon black at mass ratio of 7: 3. The CV measurements were conducted using a three-electrode half-cell using a 0.1 M Na 2 SO 4 electrolyte and a mercury sulfate electrode (MSE) as reference electrode. The CVs of carbon black show Mn 5 O 8 material is the major contributor to the overall capacitance ( Supplementary Fig. 3 ). The Mn 5 O 8 nanoparticles show a wide potential window between −1.7 V (corresponding to overpotential of 0.64 V towards HER) and 0.8 V (corresponding to overpotential of 0.63 V towards OER), demonstrating the high resistance to gas evolution reactions. To our knowledge, this is the first demonstration for a stable 2.5 V potential window in an aqueous Na-ion half-cell. Moreover, the resistive capability of the Mn 5 O 8 electrode towards HER and OER can also be demonstrated by analyzing the reaction kinetics of HER and OER using TAFEL plots ( Supplementary Fig. 4 ). The results show that Mn 5 O 8 has sluggish HER and OER kinetics, demonstrated by high TAFEL slopes at various scan rates, compared with various commercial Mn 3 O 4 and Co 3 O 4 nanopowders ( Supplementary Fig. 5 ). Figure 2: Electrochemical measurements of Mn 5 O 8 electrodes in a half-cell. ( a ) CVs show a stable potential window of 2.5 V and large overpotential ( η ) towards HER and OER. ( b ) Electro-kinetics study of CV at 500 mV s −1 . The contributions from capacitive process (blue) and diffusion-limited redox process (red) are shaded. ( c ) Capacitive contribution to the total charge stored at various scan rates in Mn 5 O 8 and Mn 3 O 4 nanoparticles and bulk materials. Full size image Figure 2a also shows nearly reversible current–voltage curves with discernable redox peaks from 1 to 1,000 mV s −1 , suggesting mixed contributions from pseudocapacitive and redox processes. There are noticeable peak shifts (blue arrows) with scan rates and peak separation between anodic and cathodic scans. The peak separation increases with scan rates but in a considerably less extent compared with battery materials. The increased peak separation is typically attributed to a higher overpotential that is required to transport the ions at faster rates. Therefore, the less-distinct peak separation here indicates that our system has the potential for high-power capability with facile Na-ion transport [6] . In addition to neutral electrolyte, CVs of Mn 5 O 8 electrodes were also conducted in Na 2 SO 4 -based electrolytes with different pH values, showing very similar behaviour in the CVs and gravimetric capacitances at the various scan rates ( Supplementary Fig. 6 ). Current–voltage relationship provides insight into the charge-storage mechanism. Assuming that the current ( i ) obeys the power law relationship with scan rate ( v ) at a given potential, and can be expressed as a combination of surface-controlled capacitive effects ( i 1 = k 1 v ) and diffusion-controlled Na-ion intercalation ( i 2 = k 2 v ½ ) (ref. 7 ): Plotting i/v ½ versus v ½ curves at a given potential, allows for the calculation of k 1 and k 2 . Thus, the contributions from capacitive charge and diffusion-limited redox charge during the CV cycling are extracted quantitatively ( Fig. 2b and Supplementary Figs 7 and 8 ). Figure 2c compares the capacitive contribution of Mn 5 O 8 nanoparticles with Mn 5 O 8 and Mn 3 O 4 bulk materials, as well as Mn 3 O 4 nanoparticles that are similar in size (18 nm) to the Mn 5 O 8 nanoparticles. Mn 3 O 4 is chosen since it has a bivalent structure (Mn 2+ Mn 3+ 2 O 4 ) analogous to that of Mn 5 O 8 (Mn 2+ 2 Mn 4+ 3 O 8 ). Figure 2c shows that Mn 5 O 8 nanoparticles have a greater contribution from capacitive storage compared with other materials. The results suggest that Mn 5 O 8 nanoparticles behave as a pseudocapacitive material due to high ratio of capacitive contribution for the charge stored, as well as its unique layered structure for facile Na-ion transport. Symmetric full cells were assembled to evaluate the electrochemical performance of Mn 5 O 8 . Each electrode was prepared by depositing Mn 5 O 8 (5 mg) and carbon black (1.25 mg) on carbon paper current collector (1.77 cm 2 ), yielding a thickness of ∼ 80 μm. With 1 M Na 2 SO 4 electrolyte, Mn 5 O 8 cell displays a stable potential window of 3.0 V after 2,000 charge and discharge cycles, the largest stable potential window ever reported for an aqueous storage device. Nearly linear potential-capacity curves, characteristic of a pseudocapacitive response, are observed ( Fig. 3a ). When current densities increase from 5 to 50 A g −1 , discharge times evolve from ∼ 42 s (corresponding to a rate of 85.7 C) to 0.75 s (a rate of 4,800 C), and electrode capacities change from 116 to 20 mAh g −1 accordingly. 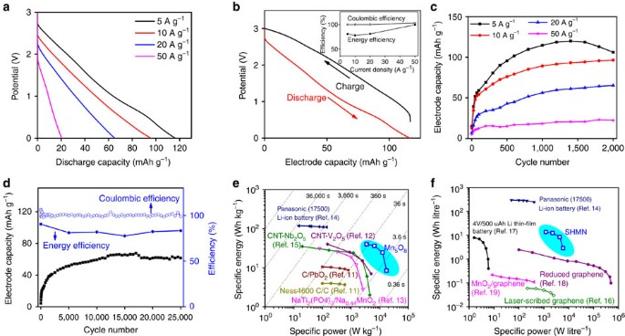Figure 3: Electrochemical tests of Mn5O8symmetric cells. (a) Discharge capacity of Mn5O8electrode as a function of current density; (b) electrode capacity during charge and discharge processes at 5 A g−1(inset: energy and coloumbic efficiencies from 5 to 50 A g−1). (c) Electrode capacity as a function of cycle; (d) Electrode capacity and coloumbic efficiencies as functions of cycle at 20 A g−1. (e) Gravimetric and (f) volumetric energy and power densities of Mn5O8cell compared with other aqueous (open symbols) and non-aqueous (solid symbols) devices. (e) Reported to the mass of electrode materials except Panasonic (17,500) Li-ion battery and Ness4600 C/C. (f) Reported to the volume of whole device. A packaging factor of 0.4 was used for Mn5O8cell since its volumetric energy and power densities are calculated based on the volume of electrode material. The results are obtained after 2,000 charge–discharge cycles unless specified otherwise. Figure 3b shows charge and discharge potential-capacity curves at various current densities ( Supplementary Fig. 9 ). The discharge curve is lower than charge curve, reflecting the charge and energy losses during cycling. Coloumbic and energy efficiencies, the ratio of the amount of charge and energy that are taken from the device versus the amount that was stored during each cycle, are shown in Fig. 3b inset after 2,000 cycles. When current density increases from 5 to 50 A g −1 , coloumbic efficiency of Mn 5 O 8 electrode remains nearly 100%, and energy efficiency increases from 80 to 97%. Figure 3c shows good cycling stability of Mn 5 O 8 full cells at a 3.0 V potential window from 5 to 50 A g −1 . At 20 A g −1 , the Mn 5 O 8 cell shows excellent coloumbic efficiency ( ∼ 100%) and energy efficiency ( ∼ 85%), and a plausible electrode capacity of 61 mAh g −1 after 25,000 cycles ( Fig. 3d ). High coulombic and energy efficiencies, good linearity between potential and electrode capacity, as well as superior cycling stability, all suggest that Mn 5 O 8 acts as a stable pseudocapacitive material at high rate. Figure 3: Electrochemical tests of Mn 5 O 8 symmetric cells. ( a ) Discharge capacity of Mn 5 O 8 electrode as a function of current density; ( b ) electrode capacity during charge and discharge processes at 5 A g −1 (inset: energy and coloumbic efficiencies from 5 to 50 A g −1 ). ( c ) Electrode capacity as a function of cycle; ( d ) Electrode capacity and coloumbic efficiencies as functions of cycle at 20 A g −1 . ( e ) Gravimetric and ( f ) volumetric energy and power densities of Mn 5 O 8 cell compared with other aqueous (open symbols) and non-aqueous (solid symbols) devices. ( e ) Reported to the mass of electrode materials except Panasonic (17,500) Li-ion battery and Ness4600 C/C. ( f ) Reported to the volume of whole device. A packaging factor of 0.4 was used for Mn 5 O 8 cell since its volumetric energy and power densities are calculated based on the volume of electrode material. The results are obtained after 2,000 charge–discharge cycles unless specified otherwise. Full size image Low-rate performance of Mn 5 O 8 cell was also studied. At low current densities, electrode capacity fades rapidly ( Supplementary Fig. 10 ). This result indicates Mn 5 O 8 acts closer to a batteries-like electrode materials at low-rate, during which storage capacity is contributed significantly from diffusion-limited redox process. This is confirmed by non-linear voltage-capacity curves at low rate, exhibiting voltage plateaus ( Supplementary Fig. 11 ), concurrent with the results obtained from CV measurements in half-cell showing that diffusion-limited redox process contributed predominately to the overall charge stored at low scan rates ( Fig. 2c ). The fact, that Mn 5 O 8 electrode capacities show an optimal performance at a current density of 5 A g −1 and fade remarkably at the low current densities (for example, 0.5 and 1 A g −1 ) in the prolonged cycles, could also be attributed to a parasitic reaction from either hydrogen or oxygen evolution occurring at low rates. The resulting gas evolution could deteriorate the Mn 5 O 8 electrode and cause the loss of capacity at prolonged cycles. It has also been pointed out that though electrode material contains Mn 3 O 4 impurity phase (<20%), it shows very sluggish electro-kinetics of HER and OER as shown in TAFEL plots and slopes ( Supplementary Figs 4 and 5 ), indicating high overpotential towards HER and OER at off-equilibrium electrochemical process at high rates. On the other hand, at low rates (0.5 and 1 A g −1 ), parasitic reaction from gas evolution, possibly catalysed by Mn 3 O 4 impurity phase, may occur in near-equilibrium condition and deteriorate the electrode materials. Mn 5 O 8 electrode materials show relatively low discharge capacities in the initial cycles, and then the capacities continuously increase before showing steady fades for the rest of the cycles. Although similar behaviours have been reported in several electrode systems [8] , [9] , [10] , the exact mechanism of the capacity increase in the initial cycling is still unclear. It has been suggested that initial cycling may help the electrode materials reach their optimal condition by facilitating the ionic transport [9] . We believe our Mn 5 O 8 electrode may undergo a similar prolonged-conditioning process during the initial cycling, reflected by the overall electrical resistance of the button-cell as calculated by i – R drop during the discharge processes. Our data show that the cell resistances decrease during the initial cycles and eventually become relatively stable and then start to increase again ( Supplementary Fig. 12 ). Correspondingly, electrode capacities show nearly opposite trends compared with cell resistances: the discharge capacities start to increase at initial cycles in a continuous manor and then show a steady fading for the rest of cycles. We have also pre-soaked the electrode materials in Na 2 SO 4 electrolyte before cell assembling in order to improve ionic transport at electrode and electrolyte interface. However, it shows that electrode capacities appear very similar trends to those shown in Fig. 3c ( Supplementary Figs 10 and 13 ). The results indicate that Na-ions transport within Mn 5 O 8 materials during the initial cycling accounts for the large cell resistance. Figure 3e shows that Mn 5 O 8 symmetric cells exhibit gravimetric energy and power densities up to 40 Wh kg −1 and 17,400 W kg −1 ; and even more impressively, exhibit volumetric energy and power densities of ∼ 13 Wh l −1 and 6,000 W l −1 ( Fig. 3f ). These values, obtained after 2,000 cycles, are much higher than those of several aqueous and even non-aqueous devices found in commercial products (less than five cycles) and recent literature in terms of gravimetric performance [11] , [12] , [13] , [14] , [15] , and volumetric performance [16] , [17] , [18] , [19] , [20] . Our Mn 5 O 8 electrode materials show very competitive performance for aqueous electrochemical energy storage especially at high rates as compared with other Mn-based electrode materials reported previously ( Supplementary Table 3 ). Further increasing the energy density of the Mn 5 O 8 electrode, especially at low current densities, will be important to develop high-performance aqueous EES devices that could rival their non-aqueous counterparts. In order to elucidate the mechanisms of this high-voltage and high-rate performance found in the Mn 5 O 8 system, we first provide synchrotron-based sXAS results with its inherent surface and elemental sensitivities, followed by the DFT calculations. First, probing the formation of interphase on the surface of Mn 5 O 8 is not trivial. As most electrode–electrolyte interphases are amorphous, STEM fails to detect the interphase layer ( Supplementary Fig. 14 ). We also carried out neutron PDF analyses on the Mn 5 O 8 nanoparticles before and after cycling in Na 2 SO 4 and D 2 O solution. Although Mn 5 O 8 nanoparticles were prepared in the heavy water (D 2 O) and tested for neutron scattering under an inert gas environment, light water (H 2 O) residuals that might be introduced from moisture in the air showed much strong scattering, so that neutron PDF analysis was unable to identify any interphase on surface of Mn 5 O 8 materials ( Supplementary Fig. 15 ). Fortunately, surface and elemental sensitivity could be achieved by synchrotron-based soft X-ray spectroscopy through the electron-decay channel [21] . In sharp contrast to neutron scattering, sXAS measurement was conducted in the ultra-high vacuum condition, so that weakly adsorbed water molecules (physically adsorbed or dissociatively adsorbed water) were completely removed and only strongly bonded molecules (for example, interphase) remained on surface. In particular, it has been well established that the hydroxyl group could be probed in water and organic molecules through oxygen K-edge sXAS, with two features at ∼ 535 and 537 eV from the unsaturated H-bonds, known as the ‘water pre-edge’ and ‘water main-peak’, respectively [22] , [23] , [24] , [25] . In addition, another post-edge hump above 540 eV is from the saturated H-bonds, especially visible in ice [23] . 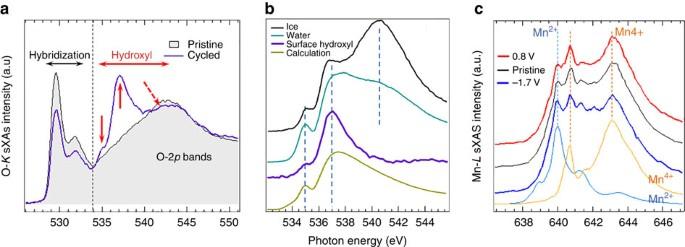Figure 4: sXAS analysis of surface hydroxylated Mn5O8. (a) O-K sXAS of Mn5O8(pristine) and Mn5O8electrode after two CV cycles between −1.7 and 0.8 V. Features below 534 eV are from the hybridization of Mn-3dand O-2pstates. The 535 and 537 eV peaks are fingerprints of the water ‘pre-peak’ and ‘main peak’. (b) A comparison of the O-K sXAS of the surface hydroxyl layer of Mn5O8with water22, ice23and one of the calculations with aligned H-bonds but lengthened O–O (3.50 and 3.00 Å) distances (Fig. 3a–gin ref.23). (c) MnL-edge of Mn5O8(pristine) and Mn5O8at different electrochemical cycling stages along with references from MnO (blue) and Li2MnO3(yellow). Figure 4a is the O-K sXAS results collected on the pristine and cycled Mn 5 O 8 electrodes with a surface probe depth of 10 nm. It is evident that, upon cycling, Mn 5 O 8 electrode displays both the fingerprinting water-features at the 535 and 537 eV. These features resemble exactly the ‘pre-edge’ and ‘main peak’ from water. Therefore, the strong spectral lineshape contrast between the pristine and the cycled electrode evidently indicates the formation of hydroxylated species on the electrode surface upon cycling. Moreover, the O–K features between 528 and 534 eV represents the spectroscopic excitations to the hybridized state of O-2 p and Mn-3 d , which are split by the crystal field of the local Mn–O coordination geometry [26] . A clear loss of intensity on this hybridization feature is observed after cycling. This intensity loss is further proof of the change of the Mn–O coordination on the surface and is consistent with the formation of hydroxyl group that covers the surface of the electrode. Figure 4: sXAS analysis of surface hydroxylated Mn 5 O 8 . ( a ) O-K sXAS of Mn 5 O 8 (pristine) and Mn 5 O 8 electrode after two CV cycles between −1.7 and 0.8 V. Features below 534 eV are from the hybridization of Mn- 3d and O- 2p states. The 535 and 537 eV peaks are fingerprints of the water ‘pre-peak’ and ‘main peak’. ( b ) A comparison of the O-K sXAS of the surface hydroxyl layer of Mn 5 O 8 with water [22] , ice [23] and one of the calculations with aligned H-bonds but lengthened O–O (3.50 and 3.00 Å) distances ( Fig. 3a–g in ref. 23 ). ( c ) Mn L -edge of Mn 5 O 8 (pristine) and Mn 5 O 8 at different electrochemical cycling stages along with references from MnO (blue) and Li 2 MnO 3 (yellow). Full size image Due to the great sensitivity of the sXAS lineshape to the hydroxyl structure, the O–K spectra reveals a very interesting molecular arrangement of the hydroxyl groups on the surface of Mn 5 O 8 electrode. Because the Mn-3 d /O-2 p hybridization features between 528 and 534 eV are purely from Mn 5 O 8 contribution, we can normalize the spectral intensity to these features and subtract the Mn 5 O 8 (pristine) signal from the after-cycling data to obtain the surface hydroxyl signal. The spectrum of the obtained surface hydroxyl signal is plotted in Fig. 4b (purple). It is clear that the surface hydroxyl layer is different from ice, missing the high energy hump from the saturated H-bonds in ice [23] . It reproduces the ‘pre-peak’ and ‘main peak’ of liquid water [22] , [23] , with the ‘main peak’ at 537.5 eV dominating the spectrum. The enhancement of this main peak has been predicted by theoretical calculations [23] , which stems from a combination of an extended O–O distance and perfectly aligned H-bonds along the O–O direction. The calculation result of the O–O distance of 3.50 Å with such a well-aligned H-bond is shown in Fig. 4b for comparison. Therefore, the O – K sXAS not only evidently shows that a hydroxyl layer is formed on the surface of the Mn 5 O 8 electrodes after cycling, it also indicates a striking ordering of the absorbed molecules, with perfectly aligned H-bonds along O–O direction, like that in ice, but with a much longer distance between the O atoms. Although the underlying mechanism of the formation of hydroxylated interphase is still unclear, we believe it is largely due to the interaction between Mn 5 O 8 surface and water during the electrochemical cycling since no hydroxylated interphase is observed in the pristine Mn 5 O 8 material ( Fig. 4a ). DFT calculations show that Mn 2+ terminated (100) surface of Mn 5 O 8 has a lower surface energy (0.87 J m −2 ) than Mn 4+ terminated (100) surface (1.80 J m −2 ). Therefore, the interaction between Mn 2+ and water during the electrochemical cycling might account for the formation of hydroxylated interphase on the Mn 2+ terminated (100) surface of Mn 5 O 8 . Second, the charge-storage mechanism is revealed by the Mn L -edge sXAS measurements ( Fig. 4c ). Mn-L sXAS is a direct probe of the Mn-3 d electron states, so the spectral lineshape is very sensitive to the normal valence of Mn [27] , [28] . Figure 4c shows the Mn L -edge sXAS data collected on the Mn 5 O 8 and the reference samples with Mn 2+ (MnO) and Mn 4+ (Li 2 MnO 3 ) valences. The spectra show that the Mn 5 O 8 electrode material is composed of Mn 4+ (641 and 643.5 eV), Mn 2+ (640 eV) and a trace amount of Mn 3+ , supporting the coexistence of Mn 5 O 8 phase and trace Mn 3 O 4 phases. The changes of peak intensity at 640 eV (Mn 2+ ), 641 eV (Mn 4+ ) and 643.5 eV (Mn 4+ ) fingerprints the evolution of oxidation states of Mn with cycling. The Mn 5 O 8 electrode at a reduced state (−1.7 V) displays a high-intensity ratio of Mn 2+ to Mn 4+ , while this ratio decreases at the oxidized state (0.8 V), suggesting the transition from Mn 2+ to Mn 4+ during oxidation processes. It is therefore evident that a two-charge transfer reaction via Mn 2+ /Mn 4+ redox couple can be achieved in the layered Mn 5 O 8 system, indicating a great potential for high-capacity energy storage. Furthermore, the mechanistic understanding of the resistive capability of surface-hydroxylated Mn 5 O 8 towards HER and OER is obtained through a comparative DFT calculation on the surfaces of hydroxylated Mn 5 O 8 , pure Mn 5 O 8 and Mn 3 O 4 . The Mn 2+ terminated (100) surface of Mn 5 O 8 is considered for the study, since our calculation predicted that Mn 2+ terminated (100) surface had a lower surface energy (0.87 J m −2 ) than Mn 4+ terminated (100) surface (1.80 J m −2 ). 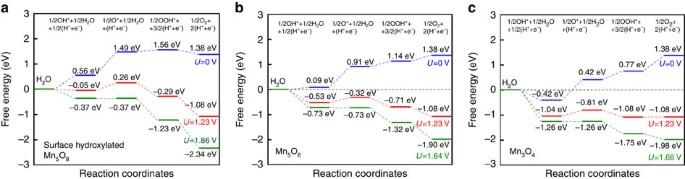Figure 5: DFT calculations. The free energy evolution for water splitting steps at different potentials on surfaces of (a) surface hydroxylated Mn5O8, (b) pure Mn5O8and (c) Mn3O4predicted from DFT. Figure 5 compares water splitting at various potential windows. Nearly all the water splitting steps are energetically unfavourable at zero potential; at a potential of 1.23 V (equilibrium potential of water splitting), all reaction steps are exothermic on three surfaces, except for OH dissociation on hydroxylated Mn 5 O 8 . The limiting potential at which all reaction steps become exothermic is determined to be 1.86, 1.64 and 1.68 V for hydroxylated Mn 5 O 8 , Mn 5 O 8 and Mn 3 O 4 , respectively, indicating hydroxylated interphase increases the energy barriers for water splitting. The activation energy of each intermediate reaction steps during the HER and OER on the three surfaces was showed ( Supplementary Fig. 16 ). The activation energy of the rate-determining step is all substantially higher for OER, indicating that OER is intrinsically difficult on all three surfaces. The activation energy of water dissociation, limiting step of HER, follows the order of hydroxylated Mn 5 O 8 (1.41 eV)>Mn 5 O 8 (0.45 eV)>Mn 3 O 4 ( ∼ 0 eV). Hydroxylated Mn 5 O 8 possesses an activation energy ∼ 1 eV higher than that of Mn 3 O 4 , implying that the reaction rate at room temperature (300 K) is at least 17 orders of magnitude slower according to the Arrhenius equation. Therefore, the DFT calculations directly support the experimental observation of high overpotential (>0.6 V) towards HER and OER for the hydroxylated Mn 5 O 8 . It was recently reported that Mn 5 O 8 nanoparticles showed very good OER activity in a neutral electrolyte in the presence of Mn 3+ species [29] . Further studies will be needed to elucidate the influence of Mn valences, such as Mn 3+ (from Mn 3 O 4 or Mn 2 O 3 phase) or Mn 2+ /Mn 4+ (from Mn 5 O 8 ), on the gas evolution reactions. Figure 5: DFT calculations. The free energy evolution for water splitting steps at different potentials on surfaces of ( a ) surface hydroxylated Mn 5 O 8 , ( b ) pure Mn 5 O 8 and ( c ) Mn 3 O 4 predicted from DFT. Full size image This work shows that an unprecedented potential window of 3.0 V in aqueous Na-ion system can be achieved through the use of surface hydroxylated Mn 5 O 8 electrodes. Gas evolution reactions are effectively inhibited through the interplay between the Mn 2+ terminated surface and hydroxylated interphase. In addition, the superior power performance of Mn 5 O 8 cell can be attributed to the unique layered, bivalence structure of Mn 5 O 8 that enables facile Na-ion transport. In general, the ion transport through the electrode and electrolyte interface is critical for the rate performance of energy storage devices. Typical approaches to mitigate the transport barrier include decreasing the dimension of electrode materials to nanoscale, designing functional layered structure for facile ion intercalation, coating secondary conductive material on electrode surface, or developing cation-disordered electrode materials with decreased energy barrier for ion transport [6] , [8] , [30] , [31] , [32] . Mn 2+ terminated (100) surface of Mn 5 O 8 has plenty of unoccupied sites, and hence provides natural tunnels for Na-ion transport along <100> direction (black arrows) ( Supplementary Fig. 17 ). Through the surface-sensitive soft X-ray spectroscopy, we also reveal the formation of a strikingly ordered ice-like surface hydroxyl layer but with much longer O–O distance after cycling. It is also possible that such a hydroxylated coating on the surface of Mn 5 O 8 modifies the interaction between Na-ion with Mn 5 O 8 by facilitating the electrostatic interaction between Na-ion and hydroxyl oxygen (red arrow). Although the electrochemical properties of Mn 5 O 8 have been largely overlooked since its structure was determined in 1965 (ref. 5 ), our result shows that Mn 5 O 8 , the only bivalence layered manganese oxide, may serve as a new generation of pseudocapacitor electrode materials for enabling a stable potential window of 3.0 V for aqueous energy storage. Our results may offer a new paradigm for developing electrode materials with a wide potential window and facile charge transfer for aqueous energy storage devices, which exhibits the performance comparable to that of non-aqueous Li-ion batteries, but much safer, less costly and more environmentally benign. In addition, it will be an interesting topic for further studies on whether and how a well ordered hydroxylated interphase could form on the surface of other metal oxides, increase their overpotential towards gas evolution reactions, and therefore increase the potential window of aqueous energy storage. Materials synthesis Synthesis was conducted in a magnetically-stirred 50 ml reaction batch of 25.3 mM MnCl 2 ·4H 2 O (Alfa Aesar, 99% metals basis) dissolved in 14 ml deionized water (DI H 2 O) (18.2 MΩ; Millipore, Inc.) at room temperature under an open environment. A 20 ml syringe was used to controllably inject a solution of 0.3 M NaOH (Alfa Aesar, 99.99% metals basis) into MnCl 2 solution at a constant flow rate of 0.167 ml min −1 for 50 min using a computer-controlled syringe pump (New Era Syringe Pumps, Inc.). The resulting dark-brown precipitate was permitted to ripen for an additional 30 min at room temperature with stirring. The product was then washed thoroughly with DI H 2 O and ethanol, vacuum-dried and then heated at 270 °C for 2 h. Electrochemical tests The anodic electrochemical properties of the Mn 5 O 8 product were studied via a three-electrode half-cell, which contained a rotating glassy carbon electrode (Pine Instrument Company) as the working electrode, a platinum wire counter electrode and mercury sulfate (saturated K 2 SO 4 ) reference electrode (MSE). The electrochemical half-cell was powered by single-channel electrochemical workstation (Model 600D, CH Instruments, Inc.). The electrode material was prepared by grinding 7 mg Mn 5 O 8 active material with 3 mg carbon black (Alfa Aesar, 99.9%) and then dissolving the mixture in DI H 2 O to a concentration of 0.5 mg ml −1 . The resulted solution was subsequently sonicated until manganese oxide was evenly dispersed in the solution and 10 μl suspension taken by pipette (Eppendorf, Inc.) was drop-cast onto the glassy carbon working electrode (0.5 cm in diameter and 0.196 cm 2 in geometric surface area). Afterwards, the working electrode was dried in vacuum with a loading of Mn 5 O 8 (3.5 μg) and carbon black (1.5 μg). Electrochemical tests were conducted in a 250 ml flat-bottom flask that contained 100 ml 0.1 M Na 2 SO 4 electrolyte (Alfa Aesar, 99.9955%) in argon-purged H 2 O with a rotating rate of 500 r.p.m. CV was conducted at voltage scan rates from 1 to 1,000 mV s −1 for six segments (three cycles) within a potential range of −1.7 to 0.8 V (versus MSE). Symmetric two-electrode button-cells were fabricated for long-term durability and stability analyses. Each electrode for full cell tests consisted of a disk (1.5 cm in diameter, 1.77 cm 2 in area) of Toray carbon paper (E-Tek, Inc.), which was coated with ∼ 5 mg Mn 5 O 8 and 1.25 mg carbon black through drop casting. The opposing electrodes were separated via cellulose-based porous filter paper (Whatman). And each button-cell contains 200 μl 1 M Na 2 SO 4 electrolyte (Alfa Aesar, 99.9955%). A stainless steel plate was placed on one side of the cell and in conjunction with a tightening bolt to ensure good electrical contact. Chronopotentiometry measurements were conducted at constant current densities from 0.5 to 50 A g −1 (with respective to each electrode for full cell measurements). Data availability The data that support the findings of this study are available from the corresponding author upon request. How to cite this article: Shan, X. et al . Bivalence Mn 5 O 8 with hydroxylated interphase for high-voltage aqueous sodium-ion storage. Nat. Commun. 7, 13370 doi: 10.1038/ncomms13370 (2016). Publisher's note: Springer Nature remains neutral with regard to jurisdictional claims in published maps and institutional affiliations.